Rapidin vivodetection of isoniazid-sensitiveMycobacterium tuberculosisby breath test There is urgent need for rapid, point-of-care diagnostic tools for tuberculosis (TB) and drug sensitivity. Current methods based on in vitro growth take weeks, while DNA amplification can neither differentiate live from dead organisms nor determine phenotypic drug resistance. Here we show the development and evaluation of a rapid breath test for isoniazid (INH)-sensitive TB based on detection of labelled N 2 gas formed specifically from labelled INH by mycobacterial KatG enzyme. In vitro data show that the assay is specific, dependent on mycobacterial abundance and discriminates between INH-sensitive and INH-resistant (S315T mutant KatG) TB. In vivo , the assay is rapid with maximal detection of 15 N 2 in exhaled breath of infected rabbits within 5–10 min. No increase in 15 N 2 is detected in uninfected animals, and the increases in 15 N 2 are dependent on infection dose. This test may allow rapid detection of INH-sensitive TB. Bacterially activated prodrugs are unusually well represented among the first- and second-line TB drugs. These include not only established drugs such as isoniazid (INH) [1] , ethionamide [2] or pyrazinamide [3] but also newly approved and developing agents such as the nitroimidazoles delamanid [4] and PA824 (ref. 5 ). The selectivity of these agents arises from their specific activation by mycobacterial enzymes, usually to reactive intermediates, and is underlined by the major mode of resistance to these agents, with mutations in genes of their activating enzymes such as katG for INH [6] , ethA for ethionamide [7] , pncA for pyrazinamide [8] and ddn for nitroimidazoles [9] . Since gene inactivation may occur through a multiplicity of single-nucleotide polymorphisms (SNPs) or insertion/deletion (indel) events, nucleic acid amplification and SNP-indel detection approaches provide only partially predictive drug susceptibility data. Beyond single-gene mutational resistance, multiple other alleles [10] , [11] , [12] , [13] , [14] and other drugs [15] , [16] may influence enzymatic activity of prodrug conversion, factors that may also limit nucleic acid-based techniques for drug susceptibility testing. Despite the importance of prodrug activation, studies have been limited to in vitro samples or bacterial culture, and at present there are no POC techniques to directly measure prodrug conversion and enzymatic activity. The mycobacterial enzyme KatG, which is responsible for INH activation, produces a range of INH-derived radicals that react with cellular components, especially the isonicotinoyl acyl radical that adds covalently to NAD + and NADP + . The adducts formed by these radicals are potent inhibitors of the key mycobacterial targets. The first target of such inhibition to be elucidated was 2-trans-enoyl-acyl carrier protein reductase (InhA) that binds INacyl-NAD + adducts, tightly inhibiting mycolic acid synthesis [17] . Although other targets or reactive species may play roles, the importance of these alternative mechanisms compared with the widely accepted inhibition of InhA remains unclear [18] . The detection of degradation products of the INacyl-NAD + adduct, such as 4-isonicotinoylnicotinamide in urine or other fluids held great promise as a measure of INH prodrug conversion in TB, and hence determining KatG activity [19] . However, this appears to lack specificity for Mycobacterium tuberculosis as 4-isonicotinoylnicotinamide was found in urine of uninfected mice treated with INH, and in urine of TB patients even when they were culture-negative after treatment [19] . Mycobacterial KatG activates INH by oxidation to a hydrazyl radical that undergoes beta scission to form isonicotinoyl acyl radical. The other product of this beta-scission reaction, diazene, has received little to no attention in the literature. To study diazene production in KatG-expressing mycobacteria, we used doubly 15 N 2 -hydrazyl-labelled INH (1) to produce doubly labelled diazene ( Fig. 1a ). Under physiologic conditions, this diazene rapidly undergoes either oxidation by unsaturated bonds ( Fig. 1b ) [20] or bimolecular disproportionation ( Fig. 1c ) to produce 15 N 2 (ref. 21 ). Diazene is widely used synthetically in the stereospecific reduction of a wide range of carbon–carbon double bonds [22] . 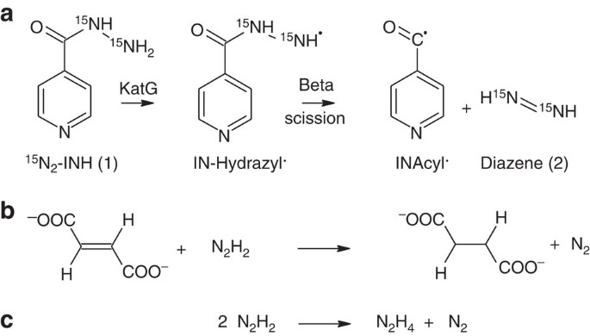Figure 1: Production of N2from KatG activation of isoniazid. (a) Production of labelled diazene from15N2-hydrazyl-labelled INH; (b) oxidation of diazene to N2by reaction with unsaturated carbon bonds such as fumarate shown, rate constant 8 × 102M−1s−1(ref.20); (c) disproportionation of diazene to N2and hydrazine rate constant 2.2 × 104M−1s−1(ref.21). Figure 1: Production of N 2 from KatG activation of isoniazid. ( a ) Production of labelled diazene from 15 N 2 -hydrazyl-labelled INH; ( b ) oxidation of diazene to N 2 by reaction with unsaturated carbon bonds such as fumarate shown, rate constant 8 × 10 2 M −1 s −1 (ref. 20 ); ( c ) disproportionation of diazene to N 2 and hydrazine rate constant 2.2 × 10 4 M −1 s −1 (ref. 21 ). Full size image This 15 N 2 produced from INH-derived diazene may be readily detected by isotope ratio mass spectrometry (IRMS), and its abundance is reported as δ 15 N 2 where Atmospheric 15 N is much lower in abundance than 14 N (~0.36%), hence 15 N 2 is very low in abundance (~13 p.p.m. ); therefore, even small amounts of 15 N 2 generation may be detected through changes in δ 15 N 2 . For example, an increase in the value of δ 15 N 2 of 250 would indicate a 25% increase in the absolute amount of 15 N 2 in a sample. This same principle is exploited by other isotope ratio breath diagnostics including the urease breath test for Helicobacter pylori infection. In this report, we describe the detection of 15 N 2 products of INH activation that are specific for mycobacterial KatG, and test their specificity against other important lung bacterial pathogens that possess related peroxidase enzymes. By measuring the increase over baseline δ 15 N 2 upon addition of the 15 N 2 -hydrazyl INH (a method termed INH→N here), we hypothesized that IRMS detection of this 15 N 2 may allow sensitive measurement of INH activation by KatG. In vitro cultures of M. tuberculosis H37Rv or M. bovis Bacillus Calmette–Guérin (BCG) were treated with 15 N 2 -hydrazyl INH in sealed tubes and portions of headspace gas collected, filtered and analysed. Treatment with 1 mg ml −1 15 N 2 -hydrazyl INH resulted in marked increases in δ 15 N 2 that were dependent upon bacterial density (CFU ml −1 ; Fig. 2a ). Next, we determined the correlation between the accumulated δ 15 N 2 and the dose of 15 N 2 -hydrazyl INH administered ( Fig. 2b ), and these experiments showed sensitive IRMS detection of headspace δ 15 N 2 following 15 N 2 -hydrazyl INH doses of 0.1 mg ml −1 , a concentration we subsequently used throughout. The generation of headspace δ 15 N 2 occurred rapidly ( Fig. 2c ), and plateau levels were reached in ~1 h. Similar data were also observed with M. bovis BCG ( Fig. 3 ), another KatG-expressing mycobacterial species, although generally lower levels of 15 N 2 production were observed compared with M. tuberculosis H37Rv. These data confirmed our ability to measure mycobacterial KatG activity quantitatively with IRMS monitoring of conversion of 15 N 2 -hydrazyl INH to 15 N 2 using in vitro cultures of mycobacteria. 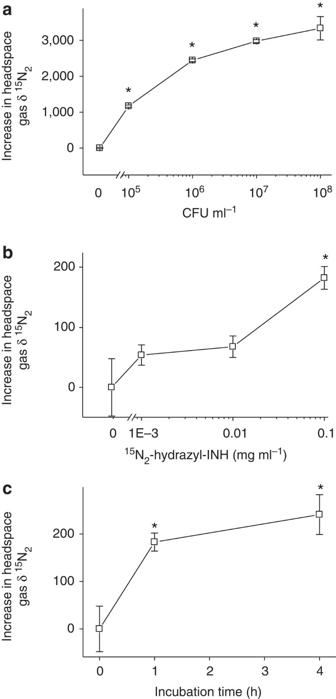Figure 2: CFU, dose and time dependence of15N2production byM. tuberculosisH37Rv. Increased headspace δ15N2(mass 30) in15N2-hydrazyl INH-treated cultures.15N2production was dependent upon (a) bacterial density ofM. tuberculosis H37Rv(3 ml) incubated with15N2-hydrazyl INH (1 mg ml−1) for 1 h, *P<0.001; (b) concentration of15N2-hydrazyl INH (H37Rv (108CFU ml−1, 3 ml) was incubated with15N2-hydrazyl INH at the indicated dose for 1 h, *P<0.001); (c) incubation time (H37Rv (108CFU ml−1, 3 ml) was incubated with15N2-hydrazyl INH (0.1 mg ml−1) for the indicated time, *P<0.001). Data represent mean±s.d. of four separate biological replicates. One-way analysis of variance (ANOVA) with Tukeypost hoctest. Figure 2: CFU, dose and time dependence of 15 N 2 production by M. tuberculosis H37Rv. Increased headspace δ 15 N 2 (mass 30) in 15 N 2 -hydrazyl INH-treated cultures. 15 N 2 production was dependent upon ( a ) bacterial density of M. tuberculosis H37Rv (3 ml) incubated with 15 N 2 -hydrazyl INH (1 mg ml −1 ) for 1 h, * P <0.001; ( b ) concentration of 15 N 2 -hydrazyl INH (H37Rv (10 8 CFU ml −1 , 3 ml) was incubated with 15 N 2 -hydrazyl INH at the indicated dose for 1 h, * P <0.001); ( c ) incubation time (H37Rv (10 8 CFU ml −1 , 3 ml) was incubated with 15 N 2 -hydrazyl INH (0.1 mg ml −1 ) for the indicated time, * P <0.001). Data represent mean±s.d. of four separate biological replicates. One-way analysis of variance (ANOVA) with Tukey post hoc test. 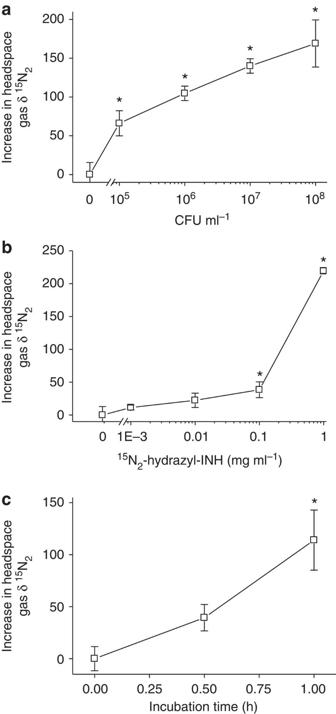Figure 3: CFU, dose and time dependence of15N2production byM. bovisBCG. Increased headspace δ5N2(mass 30) in15N2-hydrazyl INH-treated cultures was dependent upon (a) bacterial density ofM. bovisBCG (3 ml) incubated with 1 mg ml−1of15N2-hydrazyl INH for 1 h, *P<0.001; (b) concentration of15N2-hydrazyl INH (M. bovisBCG (108CFU ml−1, 3 ml) was incubated with15N2-hydrazyl INH at the indicated dose for 1 h, *P<0.001); (c) incubation time (M. bovisBCG (108CFU ml−1, 3 ml) was incubated with15N2-hydrazyl INH (1 mg ml−1) for the indicated time, *P<0.001). Data represent mean±s.d. of three separate biological replicates. One-way ANOVA with Tukeypost hoctest. Full size image Figure 3: CFU, dose and time dependence of 15 N 2 production by M. bovis BCG. Increased headspace δ 5 N 2 (mass 30) in 15 N 2 -hydrazyl INH-treated cultures was dependent upon ( a ) bacterial density of M. bovis BCG (3 ml) incubated with 1 mg ml −1 of 15 N 2 -hydrazyl INH for 1 h, * P <0.001; ( b ) concentration of 15 N 2 -hydrazyl INH ( M. bovis BCG (10 8 CFU ml −1 , 3 ml) was incubated with 15 N 2 -hydrazyl INH at the indicated dose for 1 h, * P <0.001); ( c ) incubation time ( M. bovis BCG (10 8 CFU ml −1 , 3 ml) was incubated with 15 N 2 -hydrazyl INH (1 mg ml −1 ) for the indicated time, * P <0.001). Data represent mean±s.d. of three separate biological replicates. One-way ANOVA with Tukey post hoc test. Full size image We then evaluated the specificity of our 15 N 2 -hydrazyl INH to 15 N 2 detection method for mycobacterial KatG activity. As may be seen in Fig. 4a , the common respiratory pathogens Staphylococcus aureus, Pseudomonas aeruginosa and Escherichia coli did not produce 15 N 2 when treated with 15 N 2 -hydrazyl INH. To determine whether our 15 N 2 -hydrazyl INH to 15 N 2 detection method for INH prodrug conversion was specific for the mycobacterial KatG, we tested the production of 15 N 2 using an M. tuberculosis strain harbouring a mutated KatG. This strain possessed the M. tuberculosis katG -S315T mutation that is known to profoundly decrease INH activation and result in drug resistance [6] . When compared with M. tuberculosis H37Rv, we found that the katG -S315T mutant did not produce any measurable 15 N 2 ( Fig. 4b ). 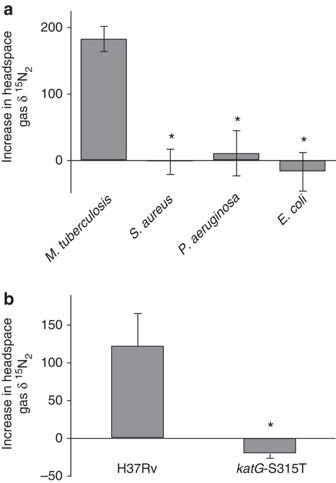Figure 4: Specificity of15N2production. (a) Increased headspace δ15N2in15N2-hydrazyl INH-treated overnight cultures ofS. aureus, P. aeruginosaandE. colicompared withM. tuberculosisH37Rv. Bacterial culture (108CFU ml−1, 3 ml) was incubated with15N-INH (0.1 mg ml−1) for 1 h. Data represent mean±s.d. (n=3 biological replicates). Student’st-test, *P<0.001. (b) Comparison in headspace δ15N2in15N2-hydrazyl INH-treated drug-sensitiveM. tuberculosisH37Rv, and an INH-resistant KatG mutant strain (katG-S315T). H37Rv orkatG-S315T strains (108CFU ml−1, 3 ml) were incubated with15N2-hydrazyl INH (0.1 mg ml−1) for 1 h. Data represent mean±s.d. (n=4 biological replicates). Student’st-test, *P<0.005. Figure 4: Specificity of 15 N 2 production. ( a ) Increased headspace δ 15 N 2 in 15 N 2 -hydrazyl INH-treated overnight cultures of S. aureus, P. aeruginosa and E. coli compared with M. tuberculosis H37Rv. Bacterial culture (10 8 CFU ml −1 , 3 ml) was incubated with 15 N-INH (0.1 mg ml −1 ) for 1 h. Data represent mean±s.d. ( n =3 biological replicates). Student’s t -test, * P <0.001. ( b ) Comparison in headspace δ 15 N 2 in 15 N 2 -hydrazyl INH-treated drug-sensitive M. tuberculosis H37Rv, and an INH-resistant KatG mutant strain ( katG -S315T). H37Rv or katG- S315T strains (10 8 CFU ml −1 , 3 ml) were incubated with 15 N 2 -hydrazyl INH (0.1 mg ml −1 ) for 1 h. Data represent mean±s.d. ( n =4 biological replicates). Student’s t -test, * P <0.005. Full size image These in vitro characteristics supported our hypothesis that the 15 N 2 -hydrazyl INH to 15 N 2, INH→N detection method might be used to detect KatG activation of INH in vivo , using a breath test approach [23] , [24] . Rabbits were infected with high dose (10 4 CFU) or low dose (10 3 CFU) M. tuberculosis H37Rv using an inhalation exposure system (Glas-col) as previously described [25] . After a 6-week incubation period, rabbits were treated with 10 mg of 15 N 2 -hydrazyl INH instilled bronchoscopically. Direct delivery to the lung was chosen to rapidly expose lung bacteria to 15 N 2 -hydrazyl INH in order to allow rapid assay, as opposed to an oral dosage form which would require absorption and redistribution. Inhaled INH has been used clinically in humans [26] . Breath samples were collected before dosing, and then at 5, 10 and 20 min post dose. Four non-infected rabbits were used as control group. It was seen that δ 15 N 2 increased rapidly in breath of all infected animals, with no observed increase in breath δ 15 N 2 of the four uninfected controls ( Fig. 5a,b ). The lack of signal in uninfected animals, together with significant signals in all infected animals, suggests that a high degree of sensitivity and specificity is inherent in this assay. Breath δ 15 N 2 reached a maximum after 5–10 min, and then variably decreased, likely because of differential distribution and absorption of 15 N 2 -hydrazyl INH from the lung into systemic circulation from the more focal pattern of delivery arising from instillation. A relationship between peak levels of δ 15 N 2 and lung CFU was observed ( Fig. 6a,b reflecting δ 15 N 2 as a function of lung CFU at the time of killing and initial infective CFU, respectively). This suggests that the approach might be sensitive to the amount of lung mycobacteria present, although significant further work is needed to delineate this relationship. Repetitive use of the technique is also likely to be complicated by the highly bactericidal nature of inhaled INH, and for monitoring of bacterial load other techniques such as urease breath tests [23] or sputum CFU may be more useful. 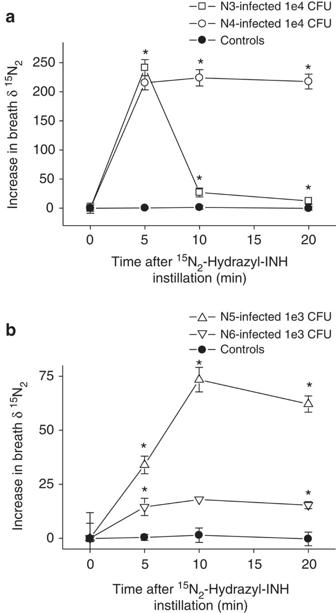Figure 5:In vivo15N2production in TB-infected and control rabbits. Increased breath in (a) high-dose- and (b) low-dose TB-infected rabbits. Rabbits were infected with high or low doses ofM. tuberculosisH37Rv, instilled with 10 mg15N2-hydrazyl INH and breath-collected. Rabbits (pathogen-free outbred New Zealand White) were infected with the indicated CFU by aerosol. At week 6, rabbits were anaesthetized with ketamine (15–25 mg kg−1) and xylazine (5–10 mg kg−1), and treated with15N2-hydrazyl INH (10 mg kg−1in 0.4 ml PBS) by intratracheal intubation. Exhaled breath gas (12 ml) was collected into Helium gas-flushed tubes at 0, 5, 10 and 20 min post15N2-hydrazyl INH administration. Data represent mean±s.d. (n=3 repeats for each rabbit N3 through N6,n=12 for four uninfected control rabbits with three repeats for each). Two-way mixed ANOVA with Bonferronipost hoctest. *P<0.001. See detailed rabbit data inTable 1. Figure 5: In vivo 15 N 2 production in TB-infected and control rabbits. Increased breath in ( a ) high-dose- and ( b ) low-dose TB-infected rabbits. Rabbits were infected with high or low doses of M. tuberculosis H37Rv, instilled with 10 mg 15 N 2 -hydrazyl INH and breath-collected. Rabbits (pathogen-free outbred New Zealand White) were infected with the indicated CFU by aerosol. At week 6, rabbits were anaesthetized with ketamine (15–25 mg kg −1 ) and xylazine (5–10 mg kg −1 ), and treated with 15 N 2 -hydrazyl INH (10 mg kg −1 in 0.4 ml PBS) by intratracheal intubation. Exhaled breath gas (12 ml) was collected into Helium gas-flushed tubes at 0, 5, 10 and 20 min post 15 N 2 -hydrazyl INH administration. Data represent mean±s.d. ( n =3 repeats for each rabbit N3 through N6, n =12 for four uninfected control rabbits with three repeats for each). Two-way mixed ANOVA with Bonferroni post hoc test. * P <0.001. See detailed rabbit data in Table 1 . 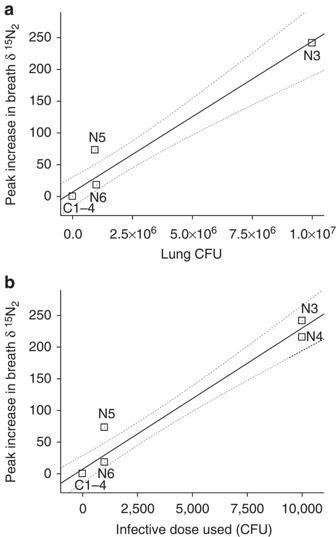Figure 6: Dependence of peak increase in breath δ15N2upon infection level. The maximal increase in breath δ15N2after15N2-hydrazyl INH delivery inFig. 5is plotted here as a function of (a) lung CFU determined at the time of killing, and (b) initial infective dose delivered. Rabbit identity numbers are shown, and 95% confidence limits are presented as dashed lines. Full size image Figure 6: Dependence of peak increase in breath δ 15 N 2 upon infection level. The maximal increase in breath δ 15 N 2 after 15 N 2 -hydrazyl INH delivery in Fig. 5 is plotted here as a function of ( a ) lung CFU determined at the time of killing, and ( b ) initial infective dose delivered. Rabbit identity numbers are shown, and 95% confidence limits are presented as dashed lines. Full size image The INH→N detection method for mycobacterial KatG activity described here is capable of discriminating between INH-susceptible and -resistant M. tuberculosis and between KatG-expressing mycobacteria and other common lung pathogens in vitro . It is also capable of rapidly discriminating between controls and animals infected with INH-susceptible TB. Potential advantages of the INH→N test are the rapid non-radioactive breath test approach, based upon detecting prodrug activation, and that samples the entire lung. The readout of this test, 15 N 2 , is detected using IRMS, and portable MS detection devices are available and under development [27] , supporting eventual development into a POC technology. Residual gas analyser MS, a technique with great potential for portability, has recently been shown to be effective in clinical IRMS [28] , and represents one avenue forward. As with any new potential diagnostic approach, ultimate clinical usage and utility must be determined in trials. Clinically, high-level INH resistance is strongly correlated to katG -S315T mutations with greatly lowered INH-activating (and INH→N) activity, whereas lower-level resistance is associated with inhA promoter mutations that will likely not be differentiated from INH-sensitive strains by the INH→N test [29] . However, INH→N assay would allow rapid point-of-care detection of katG -S315T and other katG mutations as part of a diagnostic approach, to enable rapid and optimal therapy. The potential for the INH→N method to report as a rapid and specific biomarker of mycobacterial load may provide useful tool for monitoring clinical trials and therapeutic efficacy. INH→N may also prove useful in diagnosis of some non-tuberculous mycobacteria, such as INH-sensitive M. kansasii [30] that can otherwise be challenging. However, since some peroxidases other than mycobacterial KatG enzymes bind INH (such as lactoperoxidase [31] ), further studies of specificity are planned. Similar approaches may also be extended to other TB prodrug classes so that effective and rapid detection of drug sensitivity/resistance through prodrug conversion can guide therapy. One example would be Delamanid and PA824 that are activated to bactericidal NO by mycobacterial Ddn [5] : using 15 N-nitro-PA824 would result in 15 NO·that could be directly detected in breath, or as 15 N-nitrate/nitrite in other samples such as blood or urine. This could provide rapid detection of drug activation (and hence sensitivity) in patients when conventional techniques such as MS detection of des-nitro-PA824 are difficult (Clif Barry, personal communication). This would allow optimal use of these drugs in therapy of multidrug resistant and extensively drug-resistant disease. More generally, while pathogen genotypes are rapidly determined without culture, the study of bacterial phenotypes in the host (as opposed to culture in which it can greatly change) is extremely challenging. However, the broad importance of phenotype and phenotype variance in pathogenesis is becoming increasingly appreciated, with specific examples of both growth phase-dependent [32] and stochastic [14] isoniazid-resistant phenotypes being recently elucidated. The ability to determine bacterial phenotypes through stable isotope detection of specific bacterial metabolic pathways without requiring culture could prove broadly valuable in complementing genomic approaches in studying microbiomes. Finally, it is worth noting that yet another reactive species from mycobacterial KatG activation of INH, in this case diazene, could play a role in INH action through reducing the key unsaturated mycobacterial molecules. Bacterial cultures M. tuberculosis H37Rv (H37Rv), M. bovis BCG, E. coli DH5α and P. aeruginosa PAO1 were gifts from Professor Vojo Deretic [33] , [34] , M. tuberculosis katG -S315T ( katG -S315T) was a gift from Professor Alex Pym [35] . S. aureus USA300 LAC was a gift from Professor Pamela Hall [36] . All bacterial cultures were grown at 37 °C with shaking. Mycobacterium cultures were prepared by thawing frozen stock aliquots: H37Rv and katG -S315T were grown in 7H9 Middlebrook liquid medium supplemented with oleic acid, albumin, dextrose and catalase (Becton Dickinson Inc., Sparks, MD, USA), 0.5% glycerol and 0.05% Tween 80. BCG was grown in the same culture medium omitting oleic acid. E. coli DH5α was grown overnight in LB broth (Becton Dickinson), P. aeruginosa strain PAO1 was grown overnight in LB broth supplemented with 1.76% NaCl and 1% glycerol, and S. aureus USA300 LAC was grown overnight in BBL Trypticase soybroth (Becton Dickinson). In vitro KatG assay Three millilitres of mycobacterial cultures (BCG, H37Rv or katG- S315T) were diluted as appropriate from week-old cultures, while other bacterial cultures ( P. aeruginosa, E. coli or S. aureus ) were diluted from overnight cultures. The 3-ml cultures were shaken aerobically and then were incubated with 15 N 2 -hydrazyl INH (at 0.1 mg ml −1 unless noted) in 12 ml Exetainer vials (Labco Ltd., Ceredigion, UK) for 1 h at 37 °C with shaking at 250 r.p.m. unless otherwise indicated. Collected headspace gas (1 ml) was filtered through 0.25-μ syringe filters and transferred into Helium-flushed Exetainers. Measurement of 15 N 2 conversion Sampled gas was analysed for 15 N enrichment in headspace N 2 by gas IRMS (Delta plus XL, Thermo Scientific Inc., Waltham, MA, USA). Samples were separated by GC immediately upstream of their inlet into the IRMS using a 30-m column packed with 5 Å molecular sieves operating at 60 °C and using ultrahigh purity helium as carrier gas. IRMS of the N 2 peak measured relative ratio of mass 30 15 N 2 versus mass 28 14 N 2 . Nitrogen gas of purity >99.99% (Matheson Tri-Gas, Albuquerque, NM, USA) was used as the reference gas. Animal experiments These consisted of four uninfected control rabbits, two rabbits infected at high dose (N3 and N4) and two rabbits infected at low dose (N5 and N6). Rabbits (females, 16–20 weeks old, 3.5–4 kg pathogen-free outbred New Zealand White, Robinson Services Inc., Mocksville, NC, USA) were aerosol-infected with M. tuberculosis H37Rv at either 10 3 or 10 4 CFUs using an inhalation exposure system as previously described [37] , [38] (Glas-col, Terre Haut, IN, USA). At week 6, rabbits were anaesthetized with ketamine 15–25 mg kg −1 and xylazine 5–10 mg kg −1 , and then 10 mg 15 N 2 -hydrazyl INH in 0.4-ml saline was instilled using intratracheal insertion through an endotracheal tube. To collect breath gas, a 14-French feeding tube connected to a 30-ml syringe was introduced through the endotracheal tube into the level of the carina to aspirate the exhaled air when the rabbit is breathing out. Breath gas (12 ml) was filtered with a 0.35-μ filter into Helium-flushed tubes before and after 15 N 2 -hydrazyl INH treatment at 0, 5, 10 and 20 min. 15 N 2 enrichment in breath gas was measured by IRMS. Immediately after breath testing, the animals were killed, and lung weight and CFU measured ( Table 1 . Rabbits were killed with intravenous euthasol (Virbac Corporation, Fort Worth, TX, USA). The rabbit model was chosen as it is the smallest model that enables ready endoscopic infection, instillation of INH and collection of breath. Table 1 Details of TB-infected rabbits. Full size table Ethic statement Animal work in this study was carried out in strict accordance with the recommendations in the Guide for the Care and Use of Laboratory Animals of the National Institutes of Health, the Animal Welfare Act and US federal law. The protocol was approved by the Institutional Animal Care and Use Committees at Johns Hopkins University (RB11M466). Statistical analysis All statistical analyses were performed using SPSS version 19 (SPSS Inc., Chicago, IL, USA). P values were determined using analysis of variance (ANOVA) and Student’s t -test, and values <0.05 were considered statistically significant. How to cite this article: Choi, S. W. et al. Rapid in vivo detection of isoniazid-sensitive Mycobacterium tuberculosis by breath test. Nat. Commun. 5:4989 doi: 10.1038/ncomms5989 (2014).